Direct growth of large-area graphene and boron nitride heterostructures by a co-segregation method Graphene/hexagonal boron nitride (h-BN) vertical heterostructures have recently revealed unusual physical properties and new phenomena, such as commensurate–incommensurate transition and fractional quantum hall states featured with Hofstadter’s butterfly. Graphene-based devices on h-BN substrate also exhibit high performance owing to the atomically flat surface of h-BN and its lack of charged impurities. To have a clean interface between the graphene and h-BN for better device performance, direct growth of large-area graphene/h-BN heterostructures is of great importance. Here we report the direct growth of large-area graphene/h-BN vertical heterostructures by a co-segregation method. By one-step annealing sandwiched growth substrates (Ni(C)/(B, N)-source/Ni) in vacuum, wafer-scale graphene/h-BN films can be directly formed on the metal surface. The as-grown vertically stacked graphene/h-BN structures are demonstrated by various morphology and spectroscopic characterizations. This co-segregation approach opens up a new pathway for large-batch production of graphene/h-BN heterostructures and would also be extended to the synthesis of other van der Waals heterostructures. Vertically stacked heterostructures of graphene and hexagonal boron nitride (h-BN) have recently revealed various novel properties and new phenomena [1] , [2] , [3] , [4] , [5] , which show great potential for enhancing the performance of graphene-based electronic devices [6] , [7] . Thus far, heterostructures of graphene and h-BN have been fabricated mainly by the typical mechanical cleavage and layer-by-layer transfer technique [6] , [8] , which is also used for obtaining other van der Waals heterostructures through stacking different two-dimensional crystals on top of each other [9] , [10] . However, the cleavage-and-transfer method is not suitable for industrial applications that require scalable low-cost approaches for the production of large-area heterostructures. To date, the growth of large-area graphene [11] , [12] and h-BN [13] on metal surfaces have been achieved by chemical vapour deposition (CVD) method. The graphene-on-h-BN (graphene/h-BN) or h-BN-on-graphene (h-BN/graphene) heterostructrues were obtained by stacking the CVD-grown graphene and h-BN on top of each other through the transfer process [14] , [15] . But the interfacial contamination is a big problem for the transfer approach, since the air, water [16] and hydrocarbon [8] can be easily trapped on surface. To obtain clean interface in the van der Waals heterostructures for better performance, direct growth of graphene and h-BN on top of each other is of great importance for their practical applications. Although CVD growth of h-BN/graphene [17] and graphene/h-BN [18] , [19] , [20] , [21] heterostructures have been reported recently, it is still a big challenge to obtain continuous, large-area and uniform heterostructures in wafer scale. CVD process and segregation are the two dominant methods for the large-scale growth of graphene or h-BN on metal surfaces [22] , [23] . During the CVD growth of graphene or h-BN, the surface of metal catalyst plays a key role in the decomposition of gas molecules and the nucleation of absorbed atoms. But once the metal surface is deactivated by fully covered graphene or monolayer h-BN, the decomposition and nucleation rates are greatly suppressed, which depresses the formation rate of another epitaxial layer on top of the first epitaxial layer [22] . On the other hand, segregation methods have been recently developed for the growth of large-area and high-quality graphene [24] , [25] and h-BN [26] , [27] . Different from the gas precursors used in CVD process, solid-state dissolved constituents (like B, C and N atoms) in the bulk of metals are used as precursors in the segregation method, which follows an underneath growth mode. For this reason, after the first layer is covered on the surface of metals, dissolved foreign atoms can continue to segregate from the bulk of metals to the interface between the first layer and the metal interface, forming the second layer under the first layer. Thus, the segregation method may open up a new efficient way for the growth of various van der Waals heterostructures. Here we report the direct growth of graphene/h-BN vertical heterostructures by a co-segregation method. By one-step vacuum annealing the designed growth substrates with embedded solid-state C and (B, N) sources, dissolved C and (B, N) sources sequentially segregate on the surface of metals, directly forming the large-area and continuous graphene/h-BN vertical heterostructures on the growth substrates. This co-segregation method may open up a new efficient way for the industrial preparation of large-area graphene/h-BN heterostructures. 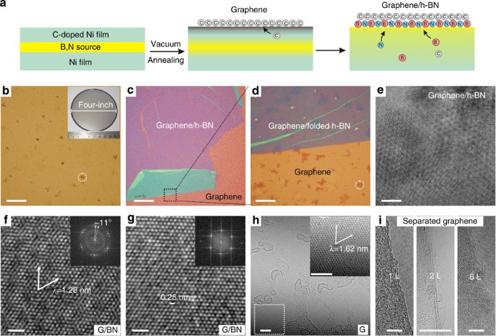Figure 1: Growth of graphene/h-BN stacked heterostructures. (a) Schematic illustration of the co-segregation growth process for graphene/h-BN heterostructures. (b) Optical image of the as-grown sample on the growth substrates. Scale bar, 20 μm. The inset is the corresponding four-inch wafer sample on the growth substrate. (c,d) Optical images of the as-grown sample transferred to a 285-nm-thick SiO2/Si substrate. Scale bars, (c) 200 and (d) 20 μm. The enlarged region of (c) that marked with dash line is shown in (d). Areas marked with dot circles in (b,d) correspond to the region with multilayer graphene. (e) TEM image of the graphene/h-BN heterostructures. Scale bar, 5 nm. (f,g) High-magnification TEM images of the graphene/h-BN heterostructures in two regions. Scale bars, 1 nm. The insets in (f,g) are the corresponding fast Fourier transform patterns. (h) Aberration-corrected HRTEM image of the separated graphene in a double-layer region. The inset is the enlarged region marked with dash line. Scale bars, 2 nm. (i) The TEM images of the separated graphene edges in three regions, revealing the thicknesses in these regions are single, two and six layers, respectively. Scale bars, 5 nm. Synthesis of graphene/h-BN heterostructures On the basis of our previous experiments on the segregation growth of individual large-area graphene [25] and h-BN [27] thin films, we specifically designed a sandwiched growth substrate for the preparation of graphene/h-BN heterostructures, as illustrated in Fig 1a . The sandwiched growth substrate is composed of a solid-state (B, N)-source embedded between a C-doped nickel (Ni) top layer and a Ni bottom layer, which are sequentially deposited on a 300-nm-SiO 2 /Si wafer substrate by electron-beam evaporations of commercial Ni, BN and C-doped Ni targets. About 2.6 at% C is included in the bulk of C-doped Ni layer [25] , and the N: B ratio is about 11% in the (B, N)-source [27] . During the vacuum annealing of the Ni(C)/(B, N)/Ni sandwiched substrates, dissolved C atoms in the bulk of C-doped Ni top layer first segregate from the bulk to the surface, nucleating and forming the graphene layer on the top of the metal surface. The B-Ni binary phase diagram shows that the B atoms can react with Ni atoms producing Ni x B ( x =1, 2, 3) compound [28] . Thus, during the annealing, B atoms in the (B, N) source and Ni atoms dissolved into each other through the reaction–diffusion process. N atoms are also brought into the bulk of Ni along with the dissolution of B atoms. When both B and N atoms diffuse to the surface of top Ni(C) layer, B and N atoms start to nucleate and grow with the form of h-BN between the graphene layer and Ni(C) surface, directly producing vertically stacked graphene/h-BN heterostructures. B and N atoms may also interdiffuse with the top graphene layer at high temperature, forming the in-plane hybrid of graphene and BN region. As shown in the inset of Fig. 1b , four-inch as-grown sample on the growth substrates can be prepared in one-time and the quantity of growth wafers is only restricted by the space of furnace, which shows great potential for mass production of large-area graphene/h-BN heterostructures. Figure 1: Growth of graphene/h-BN stacked heterostructures. ( a ) Schematic illustration of the co-segregation growth process for graphene/h-BN heterostructures. ( b ) Optical image of the as-grown sample on the growth substrates. Scale bar, 20 μm. The inset is the corresponding four-inch wafer sample on the growth substrate. ( c , d ) Optical images of the as-grown sample transferred to a 285-nm-thick SiO 2 /Si substrate. Scale bars, ( c ) 200 and ( d ) 20 μm. The enlarged region of ( c ) that marked with dash line is shown in ( d ). Areas marked with dot circles in ( b , d ) correspond to the region with multilayer graphene. ( e ) TEM image of the graphene/h-BN heterostructures. Scale bar, 5 nm. ( f , g ) High-magnification TEM images of the graphene/h-BN heterostructures in two regions. Scale bars, 1 nm. The insets in ( f , g ) are the corresponding fast Fourier transform patterns. ( h ) Aberration-corrected HRTEM image of the separated graphene in a double-layer region. The inset is the enlarged region marked with dash line. Scale bars, 2 nm. ( i ) The TEM images of the separated graphene edges in three regions, revealing the thicknesses in these regions are single, two and six layers, respectively. Scale bars, 5 nm. Full size image Morphology and structure characterizations Figure 1b shows the optical image of as-grown samples. The dark region marked with dashed circle is quite similar with the morphology of CVD-grown multilayer graphene islands on metals [12] . To confirm the stacked heterostructures, the as-grown samples on the wafer-scale substrates were cut into small pieces and transferred to different substrates using the poly (methyl methacrylate) (PMMA)-mediated transfer-printing technique [12] . Because the h-BN layers in the heterostructures are not directly adhered to the supported PMMA layer during the transfer process, h-BN layers underneath the top graphene layers can be folded and scratched away with the assistance of low-power sonication or other mechanical force, producing separated graphene layer and graphene/h-BN heterostructures (see Supplementary Fig. 1 ). As shown in Fig. 1c,d , the large-area graphene/h-BN heterostructures transferred onto the 285-nm-thick SiO 2 /Si substrates can be clearly identified from the separated graphene layer by the colour contrast in the optical images. Figure 1d illustrates the enlarged image of the dash line marked region in Fig. 1c , which shows that graphene is continuous across the edge between the graphene/folded-h-BN and the separated graphene. By controlling the transfer process, the h-BN layers can be remained or fully removed, leaving the complete graphene/h-BN heterostructures or isolated graphene layer for other characterizations. As shown in Fig. 1e–g , high-resolution transmission electron microscopy (TEM, FEI F30, operated at 300 kV) was used to examine the microstructure of the graphene/h-BN heterostructures. Free-standing graphene/h-BN heterostructures was transferred onto TEM grids. As shown in Fig. 1e,f , clear Moiré patterns are observed in the high-resolution TEM images of the complete graphene/h-BN heterostructures. As shown in Fig. 1f , the Moiré pattern wavelength is measured to be about 1.28 nm, and the fast Fourier transform pattern of Fig. 1f displays two sets of hexagonal spots with a rotation angle about 11° (inset of Fig. 1f ). As the lattice mismatch between graphene and h-BN (~1.8%) is very small, the Moiré pattern can be ascribed to the rotation between the graphene lattice and h-BN lattice [3] or the rotation between two kind of h-BN lattice or graphene lattice. As shown in the inset of Fig. 1g , only one set of hexagonal spots is distinguished, which suggests that the rotation angle between graphene and h-BN is close to 0° in the examined region ( Fig. 1g ). Figure 1g demonstrates that the hexagonal lattice spacing is about 0.25 nm, which is close to the h-BN lattice constant (0.250 nm) and graphite lattice (0.246 nm) [23] . After removing the bottom h-BN layers in the vertical heterostructures, the separated graphene were transferred onto TEM grids for TEM characterization, as shown in Fig. 1h,i and Supplementary Fig. 2 . Spherical aberration-corrected TEM (FEI 80–300 environmental Titan (S) TEM, operated at 80 kV) was taken on the separated graphene to achieve its high-resolution TEM images. Figure 1h shows the aberration-corrected HRTEM image of a double-layer region of the separated graphene, which reveals the Moiré patterns with a wavelength about 1.62 nm (inset of Fig. 1h ). By observing folded edges of the separated graphene in TEM images, most of the observed regions are found to be single layer ( Fig. 1i ). Some double-layer and multilayer graphene regions are also observed ( Fig. 1i ), which are consistent with the multilayer regions marked with dot circle in Fig. 1b,d . The corresponding scanning electron microscopy images (see Supplementary Fig. 3 ) and atomic force microscopy images (see Supplementary Fig. 4 ) also reveal that most of the regions in the separated graphene are single to few-layer graphene and multilayer graphene regions are sporadic distributed. X-ray photoelectron spectroscopy characterization X-ray photoelectron spectroscopy (XPS) was taken to determine the vertically stacked graphene/h-BN heterostructures grown on the surface of the growth substrates, since XPS is a surface-sensitive technique that can collect the signals of electrons escaping from the top 0 to about 10 nm in depth of the test materials. As shown in Fig. 2a,b , the B1s peak and N1s peak are located at ~190.1 eV and ~397.7 eV respectively, which are in good agreement with the standard XPS values for h-BN [13] , [27] . The N:B atomic ratio calculated from the XPS data is about 1.01:1, which is close to the 1:1 ratio in h-BN. As shown in Fig. 2c , the C1s peak at 284.8 eV corresponds to the C–C bonding in graphene or graphite. Small N1s peak at 400.1 eV and C1s peak at 288.6 eV are also observed in Fig. 2b,c respectively, reflecting the presence of bonding between N and C atoms [29] , [30] . The N–C bonds indicate that the in-plane hybridization of graphene and h-BN may also exist in the heterostructures [30] . As illustrated in Fig. 2d , XPS depth-profiling examinations are taken on the samples grown on the growth substrates, and the Ar-ion etching rate is about 0.3 nm per 18 s basing on the calibration of Ni. As shown in Fig. 2e,f , the intensities of N1s and C1s decrease as the etching depth increases, indicating the heterostructures are gradually removed by etching. The peak positions of N1s do not change as the etching depth increases, which indicate the same N-B chemical state in the etched depth. On the other hand, the positions of C1s peaks gradually shift from 284.8 to 283.7 eV. The lower binding energy of C1s at 283.7 eV corresponds to the individual C atoms dissolved in Ni [31] . Thus, the observed intensity of C1s comes from two parts: C atoms in graphite and the individual C atoms dissolved in Ni. After etching the top 0.3 nm of the samples, the intensity of C1s decreases sharply ( Fig. 2f ); however, the intensity of N1s is almost of no change ( Fig. 2e ), which agrees well with the construction of vertically stacked graphene-on-h-BN heterostructures. From 0 to 0.6 nm depth, the integrated intensity (area) of the N1s is almost of no change, while that of C1s decreases sharply (see Supplementary Fig. 5 ), which supports the vertical stacked graphene-on-h-BN structure. The follow-up decrease of C1s peak is ascribed to the etching of sporadic multilayer graphene islands. 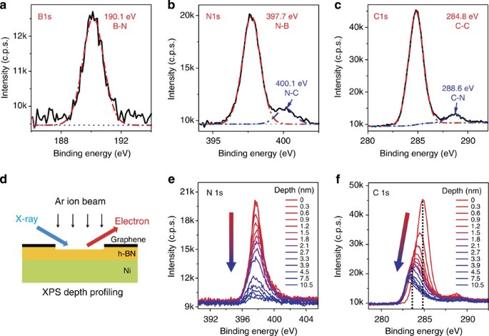Figure 2: XPS characterizations of the graphene/h-BN heterostructures. (a) B1s (b) N1s (c) C1s peaks of the samples on the growth substrates. (d) Schematic of the XPS depth-profiling process. (e,f) Evolution of N1s and C1s peaks as a function of the etching depth. Figure 2: XPS characterizations of the graphene/h-BN heterostructures. ( a ) B1s ( b ) N1s ( c ) C1s peaks of the samples on the growth substrates. ( d ) Schematic of the XPS depth-profiling process. ( e , f ) Evolution of N1s and C1s peaks as a function of the etching depth. Full size image Other spectroscopic characterizations To further demonstrate the presence of graphene and h-BN in the heterostructures, Raman and ultraviolet–visible absorption spectroscopy were taken to characterize the transferred samples. 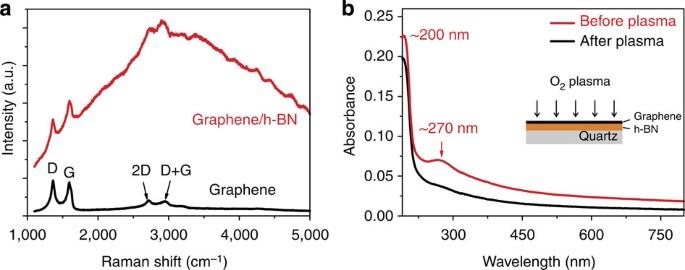Figure 3: Spectroscopic characterizations of the graphene/h-BN heterostructures. (a) Raman spectra in the graphene/h-BN and separated graphene regions. (b) Ultraviolet–visible absorption spectroscopy of the graphene/h-BN before and after plasma etching. The inset shows the plasma etching process. Figure 3a shows the Raman spectra recorded on the regions of graphene/h-BN and separated graphene (as indicated in Fig. 1c ). The typical peaks of graphene, such as D (~1,363 cm −1 ), G (~1,593 cm −1 ), 2D (~2,714 cm −1 ) and D+G (~2,958 cm −1 ), are displayed in both the graphene/h-BN and separated graphene regions, indicating the presence of graphene in the heterostructures [32] . Raman mapping of the separated graphene is also used to identify the multilayer graphene islands (see Supplementary Fig. 6 ). As the overlapping of D peak in the top graphene and the strong photoluminescence background, the Raman peak of h-BN at ~1,370 cm −1 is not clearly identified in the graphene/h-BN ( Fig. 3a ). As shown in the optical images of the transferred samples before and after plasma etching (see Supplementary Fig. 7 ), the graphene layer can first be removed from the vertical graphene/h-BN heterostructures. After the graphene layer is removed, the representative optical phonon of h-BN at 170 meV (ref. 33 ) (corresponding to a wavenumber of ~1,370 cm −1 ) is clearly identified by the Raman and photoluminescence spectra of the isolated h-BN in the heterostructures (see Supplementary Fig. 8 ). The photoluminescence background displayed in graphene/h-BN region can be ascribed to the defect states of h-BN such as line defects along the grain boundaries [27] , [34] . For the as-grown samples transferred to quartz substrates, the ultraviolet–visible absorption spectrum shows two peaks at ~200 and ~270 nm ( Fig. 3b ), which describe the optical bandgap of h-BN [27] and the excitonic effects in graphene [35] . After plasma etching (inset of Fig. 3b ), the graphene excitonic peak at ~270 nm disappears, indicating the remove of the top graphene layer in the vertical graphene-on-h-BN heterostructures. Figure 3: Spectroscopic characterizations of the graphene/h-BN heterostructures. ( a ) Raman spectra in the graphene/h-BN and separated graphene regions. ( b ) Ultraviolet–visible absorption spectroscopy of the graphene/h-BN before and after plasma etching. The inset shows the plasma etching process. Full size image Auger electron spectroscopy (AES) was also taken to investigate the graphene/h-BN and separated graphene regions of the samples transferred on SiO 2 /Si substrate. In comparison with XPS, AES is more surface sensitive, whose signals are mainly from the top layers. As shown in Fig. 4a , only B(KLL), C(KLL), N(KLL), O(KLL), Si(KLL) signals are observed in the spectra of the two regions. The C signals are mainly from the graphene, while B and N are from the h-BN layers. The Si and O signals are from the SiO 2 /Si substrate. For the separated graphene region, the presence of B and N signals indicates the in-plane hybridization of graphene and h-BN, which are in accordance with our observation of N–C bond in the XPS results and the D peak in Raman. AES depth-profile examination is also taken on the transferred samples, and the sputtering rate is about 0.3 nm min −1 based on the calibration of SiO 2 . 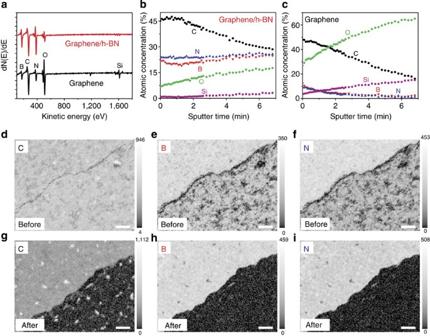Figure 4: Auger electron spectroscopy and elemental mapping of the graphene/h-BN heterostructures. (a) Auger electron spectroscopy of the graphene/h-BN and separated graphene regions. (b,c) Atomic concentration evolutions of C, N, B, O and Si during sputtering for the graphene/h-BN and isolated graphene regions, respectively. The etching rate is about 0.3 nm min−1based on the calibration of SiO2. (d) C, (e) B and (f) N mapping of the transferred samples near the boundary of graphene/h-BN (upper left region) and separated graphene (lower right region) before plasma etching. (g) C, (h) B and (i) N mapping of the transferred samples near the boundary of graphene/h-BN (upper left region) and separated graphene (lower right region) after plasma etching. Scale bars ind–i, 5 μm. Figure 4b,c displays the evolution of atomic concentration of C, N, B, O and Si for the graphene/h-BN and separated graphene regions, respectively. As sputtering time increases, the C concentrations in the two regions both decrease, indicating the top graphene layer in the heterostructure is firstly etched. The B and N atoms doped in graphene are also etched away as sputtering time increases ( Fig. 4c ). And the increase of Si and O concentration also agrees with the etching of top graphene layer. However, the B and N concentrations in graphene/h-BN remain the same as sputtering time increases ( Fig. 4b ), indicating the h-BN underneath the graphene layer is not etched firstly. These AES results agree well with the construction of graphene-on-h-BN heterostructures. Figure 4: Auger electron spectroscopy and elemental mapping of the graphene/h-BN heterostructures. ( a ) Auger electron spectroscopy of the graphene/h-BN and separated graphene regions. ( b , c ) Atomic concentration evolutions of C, N, B, O and Si during sputtering for the graphene/h-BN and isolated graphene regions, respectively. The etching rate is about 0.3 nm min −1 based on the calibration of SiO 2 . ( d ) C, ( e ) B and ( f ) N mapping of the transferred samples near the boundary of graphene/h-BN (upper left region) and separated graphene (lower right region) before plasma etching. ( g ) C, ( h ) B and ( i ) N mapping of the transferred samples near the boundary of graphene/h-BN (upper left region) and separated graphene (lower right region) after plasma etching. Scale bars in d – i , 5 μm. Full size image To visualize the structure of graphene/h-BN heterostructures as displayed in Fig. 1c , AES elemental mapping ( Fig. 4d–i ) was taken on the transferred samples near the boundary region of graphene/h-BN (upper left regions of Fig. 4d–i ) and separated graphene (lower right regions of Fig. 4d–i ). As shown in Fig. 4d , the intensity distribution of C before plasma etching is nearly the same in the graphene/h-BN and separated graphene region, indicating the graphene is the first top layer in the vertical heterostructure. But for B and N mapping before plasma etching, the intensities in graphene/h-BN region are stronger than that in separated graphene region ( Fig. 4e,f ). After the first top 2 nm is etched away by Ar-ion (same process as Fig. 4b,c ), the C ( Fig. 4g ), B ( Fig. 4h ) and N ( Fig. 4i ) intensities in the previous separated graphene region are close to zero. The white dots shown in Fig. 4g are the residual multilayer graphene layers. Some residual C still exists in the previous graphene/h-BN region ( Fig. 4g ), which may be ascribed to the carbon doped in h-BN layer or the etching rate difference on SiO 2 and h-BN substrates (see Supplementary Fig. 9 ). The B and N elements only exist in the previous graphene/h-BN region after plasma etching ( Fig. 4h,i ), indicating the h-BN layers are under the top graphene layer in the vertical heterostructure. By removing the bottom h-BN layers in the transfer process, the top graphene layer in the heterostructures can be completely separated for further characterizations. Fig. 5a shows the optical image of the large area separated graphene transferred on SiO 2 /Si substrate. The ultraviolet–visible absorption spectrum of the separated graphene transferred on quartz also displays two characteristic peaks at ~200 and ~270 nm ( Fig. 5b ), which indicates the presence of h-BN and graphene domains [30] . The bonding between N and C atoms shown in XPS ( Fig. 2b,c ), D peak in the Raman ( Fig. 3a ) and B, N signals in the AES of the separated graphene ( Fig. 4a ) also reveal the in-plane hybridization of h-BN and graphene domains for our separated samples, as illustrated in the inset of Fig. 5b . For our co-segregation method, the hybridization of h-BN and graphene domains may ascribe to the interdiffusion between B, N and C atoms in the high-temperature growth process, which is also a general phenomenon for the CVD growth of stacked heterostructures of graphene and h-BN [17] , [20] . 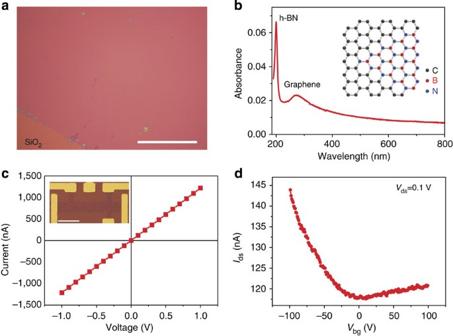Figure 5: Characterizations of the separated grapheme. (a) Optical image of the large-area separated graphene film. Scale bar, 500 μm. (b) Ultraviolet–visible absorption spectroscopy of the separated graphene film transferred on quartz. The characteristic two peaks at ~200 and ~270 nm indicates the presence of h-BN and graphene domains. The inset is the schematic structure of the separated graphene. (c)I–Vcurve of the separated graphene. Inset is the optical image of the device and the scale bar is 40 μm. (d) The source-drain current (Ids) as a function of the back gate voltage (Vbg) for the separated graphene, and the source-drain voltage (Vds) is 0.1 V. Figure 5: Characterizations of the separated grapheme. ( a ) Optical image of the large-area separated graphene film. Scale bar, 500 μm. ( b ) Ultraviolet–visible absorption spectroscopy of the separated graphene film transferred on quartz. The characteristic two peaks at ~200 and ~270 nm indicates the presence of h-BN and graphene domains. The inset is the schematic structure of the separated graphene. ( c ) I – V curve of the separated graphene. Inset is the optical image of the device and the scale bar is 40 μm. ( d ) The source-drain current ( I ds ) as a function of the back gate voltage ( V bg ) for the separated graphene, and the source-drain voltage ( V ds ) is 0.1 V. Full size image Recent theoretical and experimental studies on the in-plane hybridization of h-BN and graphene have revealed various novel tunable magnetic and electronic properties of this hybrid material [36] , [37] . To investigate the influence of the in-plane hybridization on the electrical transport properties, back-gated field-effect transistors of the separated graphene were fabricated on 285-nm-thick SiO 2 /Si substrates by optical lithography and following electrode deposition techniques (inset of Fig. 5c ). The linearly current–voltage ( I – V ) curve of the separated graphene reveals its conducting nature ( Fig. 5c ). Because of the BN domains hybridized in the graphene lattice, the sheet resistance of the separated graphene ( R s = R · W / L ~200 kΩ per sq) is approximately three orders of magnitude higher than the pristine CVD-grown graphene [12] . Figure 5d shows the source-drain current ( I ds ) as a function of the back gate voltage ( V bg ) at the 0.1 V source-drain voltage ( V ds ). The I ds – V bg curve of the separated graphene shows an ambipolar semiconducting behaviour, which is similar to that of pristine CVD-grown graphene [12] . The carrier mobility is calculated to be about 1.5 cm 2 V −1 s −1 , which is at the same level of the CVD-grown in-plane-hybridized graphene-BN films [30] . Because the carrier mobility of the separated graphene is still low at present, no enhanced electrical performance is shown in the graphene-on-h-BN heterostructrues (see Supplementary Fig. 10 ). However, a recent study shows that good control on the domain size and relative concentration of graphene and h-BN domains can improve their carrier mobility and on/off ratio [37] . Thus, our samples are still needed to further control on the in-plane hybridization of graphene and h-BN domains to achieve better performance. In our co-segregation method, the annealing temperature and the structure of Ni(C)/(B, N)/Ni sandwiched growth substrate are the two key controlling parameters. The diffusion rates of dissolved B, N and C atoms increase as the temperature increases. Thus, the amount of B and N atoms that diffuse to the metal surface increase as temperature increases for the same given time, which can be used to control the thickness of the underneath h-BN layers in the heterostructures (see Supplementary Fig. 11 ). By increasing the heating temperature from 950 to 1,000 and 1,050 °C, the thickness of h-BN increase from 10 to 16 and 25 nm (see Supplementary Fig. 12 ). The coverage and size of multilayer graphene islands decrease as temperature increases (see Supplementary Fig. 13 ), because the carbon solubility in Ni bulk increases as temperature increases [28] . As the carbon atoms for segregated graphene are from Ni(C) layer, the graphene growth shows great dependence on thickness of Ni(C) (see Supplementary Fig. 14 ). Thicker Ni(C) lead more carbon to form multilayer graphene islands, while graphene cannot be formed when the Ni(C) is too thin to supply the carbon amount for the growth of monolayer graphene (see Supplementary Fig. 14 ). Our previous work on the segregation growth of h-BN has shown that the thickness of (B, N) source is also an important parameter for controlling the thickness of h-BN [27] . Our controllable experimental design on the co-segregation growth of graphene/h-BN heterostructures may be extended to other van der Waals heterostructures by designing new sandwiched growth substrates with other dissolved foreign atoms, such as Mo(S)/(B, N)/Ni growth substrates to get vertical heterostructure of MoS 2 and h-BN. In summary, we have developed a novel co-segregation method to realize the direct growth of wafer-scale vertically stacked graphene/h-BN heterostructures. C and (B, N) source dissolved in the Ni(C)/(B, N)/Ni sandwiched growth substrates can be sequentially segregated on the metal surface by vacuum annealing, directly forming the graphene top layer and h-BN under layers. The vertically stacked van der Waals heterostructures were confirmed by various morphology and spectroscopic characterizations. The graphene top layer in the heterostructure can be separated for characterizations, which demonstrates the actually in-plane hybridization structure. This work opens up a new way for mass production of large-area vertically stacked graphene/h-BN heterostructures and other van der Waals heterostructures. Preparation of growth substrates The Ni film (400 nm), (B, N) source (60 nm) and carbon-doped Ni film (150 nm) are sequentially deposited on four-inch 300-nm-thick SiO 2 /Si wafer substrates using electron beam evaporator (ULS400, Balzers, pressure 1 × 10 −5 Pa before evaporation), forming sandwiched growth substrates Ni(C)150 nm/(B, N) 60 nm/Ni 400 nm/SiO 2 /Si. The weight purities of the commercial Ni and BN targets are 99.99%. The carbon weight in the carbon-doped Ni target is ~1 wt %. The working pressure for Ni and carbon-doped Ni evaporation is 1–3 × 10 −5 Pa, while the working pressure for (B, N) source is 10 −2 –10 −1 Pa because of the decomposition of BN during the evaporation process. Growth procedures The sandwiched Ni(C)/(B, N)/Ni samples were loaded into the vacuum annealing furnace (VTHK-350, Beijing Technol Science Co.) for annealing. After the furnace was evacuated to ~5 × 10 −5 Pa, the samples were heated to desired temperatures (950, 1,000 and 1,050 °C) at a rate of 20 °C min −1 and maintained at the desired temperatures for 10 min at a working pressure of 10 −3 –10 −4 Pa. Then the samples were cooled down to room temperature naturally at a rate of 2–50 °C min −1 after the heater power was shut down. The graphene/h-BN heterostructures films can be detached from the growth substrates and transferred to target substrates using the typical PMMA–mediated transfer-printing technique [12] . All the data are collected on samples with three desired heating temperature at 950, 1,000 and 1,050 °C: Fig. 1 and Raman data in Fig. 3a are taken on sample-950 °C; XPS data in Fig. 2 and ultraviolet–visible data in Fig. 3b are taken on sample-1,000 °C; Fig. 4 and Fig. 5 are taken on sample-1,050 °C. Characterizations We characterized our samples by optical microscopy (Olympus BX51), TEM (FEI F30 operated at 300 kV; spherical aberration-corrected FEI 80–300 environmental Titan (S) TEM, operated at 80 kV), atomic force microscopy (Veeco nanoscope, tapping mode), scanning electron microscopy (Hitachi S-4800, 1kV), XPS (AXIS-Ultra), Raman spectroscopy (Horiba HR800, 457.9 nm, 2 mW), ultraviolet–visible absorption spectroscopy (Lambda 950), AES (PHI-700) and electrical measurements (Keithley, SCS-4200). How to cite this article : Zhang, C. et al . Direct growth of large-area graphene and boron nitride heterostructures by a co-segregation method. Nat. Commun. 6:6519 doi: 10.1038/ncomms7519 (2015).